Elfn1 recruits presynaptic mGluR7 in trans and its loss results in seizures GABAergic interneurons are highly heterogeneous, and much is unknown about the specification and functional roles of their neural circuits. Here we show that a transinteraction of Elfn1 and mGluR7 controls targeted interneuron synapse development and that loss of Elfn1 results in hyperactivity and sensory-triggered epileptic seizures in mice. Elfn1 protein increases during postnatal development and localizes to postsynaptic sites of somatostatin-containing interneurons (SOM-INs) in the hippocampal CA1 stratum oriens and dentate gyrus (DG) hilus. Elfn1 knockout (KO) mice have deficits in mGluR7 recruitment to synaptic sites on SOM-INs, and presynaptic plasticity is impaired at these synapses. In patients with epilepsy and attention deficit hyperactivity disorder (ADHD), we find damaging missense mutations of ELFN1 that are clustered in the carboxy-terminal region required for mGluR7 recruitment. These results reveal a novel mechanism for interneuron subtype-specific neural circuit establishment and define a common basis bridging neurological disorders. GABAergic interneurons in the mammalian neocortex constitute a relatively small population in comparison to excitatory neurons, but are highly heterogeneous [1] . Recent studies have defined the properties of interneuron subtypes based on their morphology, functionality, molecular markers and origins [2] , [3] . Although interneurons are known to participate in local neural circuits in a subtype-specific manner, the molecular basis by which the connectivity of each interneuron is determined remains unclear. Furthermore, although GABAergic interneurons are proposed to be essential for excitatory and inhibitory balance [4] , little is known of the behavioural and physiological pathology caused by the genetic dysfunction of neural circuitry that contains specific local interneurons. Hippocampal interneurons are appropriate for addressing these issues because of their distinct and relatively well-characterized properties. Among them, oriens lacunosum moleculare (OLM) cells in the CA1 region and hilar perforant path-associated (HIPP) cells in the DG share the following features: they (1) innervate the distal dendrites of principal neurons (CA1 pyramidal neurons and DG granule neurons); (2) fire rhythmically at theta frequency [5] , [6] ; (3) co-express somatostatin (SOM), neuropeptide Y and metabotropic glutamate receptor 1a (mGluR1a) [7] , [8] , [9] ; and (4) are decorated by metabotropic glutamate receptor 7 (mGluR7)-containing presynaptic structures [10] , [11] . Furthermore, both OLM and HIPP cells are affected in several models of temporal lobe epilepsy, suggesting the clinical importance of this subset of interneurons [12] , [13] . The presynaptic mGluR7 in local circuits involving OLM and HIPP cells is considered to control brain excitability and higher cognitive function [14] , [15] , [16] , [17] . mGluR7 exists in the presynaptic active zone, and interestingly, the protein is differentially concentrated at the single synaptic terminal, depending on the nature of the postsynaptic neurons [10] . This finding suggests that some key molecules on OLM/HIPP cells trigger presynaptic mGluR7 accumulation. mGluR7 binds to the presynaptic scaffold protein PICK1 through its C terminus, and this interaction is essential for its presynaptic clustering [18] , [19] and suppression of seizures [15] , [16] . However, binding to PICK1 alone cannot explain the accumulation of mGluR7 onto specific interneurons. Although mGluR1a would seem to be a candidate postsynaptic determinant, this is not the case. The absence of mGluR1a does not affect the high level of mGluR7 [10] , suggesting the existence of an as-yet-unidentified molecule. Here we show that the transmembrane protein Elfn1 (extracellular-leucine-rich repeat (LRR) fibronectin domain1) [20] in OLM cells is a critical postsynaptic component that induces mGluR7-positive presynaptic structures in excitatory neurons. The neurological phenotypes we observed in Elfn1 knockout (KO) mice are strikingly similar to those of mGluR7-deficient mice, suggesting that the functions of Elfn1 and mGluR7 proteins are closely linked. Furthermore, in searching for ELFN1 variants in patients with neurological disorders, we identified novel missense mutations that specifically impair the mGluR7-recruiting function of ELFN1 via its C-terminal domain. These findings raise the possibility that dysfunction of the ELFN1–mGluR7 complex is a critical contributor to neurological diseases. Elfn1 localizes to excitatory postsynapses on SOM-INs Elfn1 is a presumptive type I transmembrane protein containing a LRR domain, a fibronectin type-III domain and a transmembrane domain ( Fig. 1a ) [20] . In mice, Elfn1 is strongly expressed in interneurons of the hippocampus (hp) and cerebral cortex [20] . 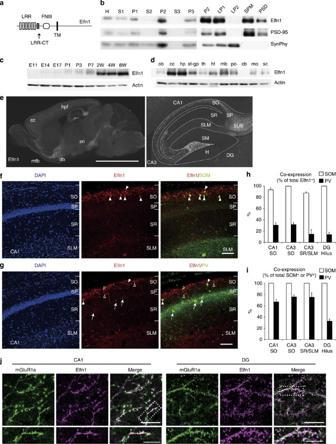Figure 1: Structure and expression of Elfn1. (a) Domain structure of Elfn1. LRR, leucine rich repeat; CT, C-terminal domain; FNIII, fibronectin type-III domain; TM, transmembrane domain. (b) Subcellular distribution of Elfn1 in the mouse brain. H, homogenates; S1, postnuclear supernatant; P1, nuclear pellet; S2, supernatant after P2 precipitation; P2, crude synaptosomes; S3, cytosol; P3, light membrane; LP1, crude synaptosomal membranes; LP2, synaptic vesicle-enriched fraction; SPM, synaptosomal plasma membranes. (c,d) Developmental expression patterns (c) and regional distribution (d) of Elfn1 protein in mouse brain as analysed by IB. P, postnatal day; W, weeks. ob, olfactory bulb; cc, cerebral cortex; hp, hippocampus; st-gp, striatum and globus pallidus; th, thalamus; ht, hypothalamus; mb, midbrain; po, pons; cb, cerebellum; mo, medulla oblongata; sc, spinal cord. Equal amounts of protein were loaded. (e) Immunofluorescence staining of Elfn1 in a frozen sagittal section of adult mouse brain. cc, cerebral cortex; hpf, hippocampal formation; mfb, magnocellular basal forebrain; db, diagonal band; sn, substantia nigra. The picture at right is a magnified view of the hippocampal formation in the picture at left. SUB, subiculum; SP, stratum pyramidale; SR, stratum radiatum; SLM, stratum lacunosum moleculare; SM, stratum moleculare; H, hilus. Scale bar, left, 5 mm. (f–i) Double immunofluorescence staining of vibratome coronal sections through the dorsal hp from 4-month-old WT mouse brain with anti-Elfn1 (red) and anti-somatostatin (f, green, SOM) or anti-PV (g, green). Scale bars, 100 μm. (h) Percentage of double-labelled neurons as a proportion of total Elfn1-positive neurons in the respective layers. (i) Percentage of double-labelled neurons as a proportion of the total number of cells immunopositive for SOM or PV. Data were obtained from one hemicoronal section per animal (n=3 mice). Mean values±s.e.m. are shown. (j) Double immunofluorescence staining of the hippocampal CA1 and DG regions. Vibratome coronal sections from 4-month-old WT mouse brain were stained with anti-Elfn1 (magenta) and anti-mGluR1a (green). Images at bottom are magnified images of the boxed regions in the upper image. Closed arrowheads and arrows, Elfn1+ and PV+ soma; open arrowheads, Elfn1+ and PV− soma. Scale bars, 20 μm for upper images and 10 μm for bottom images. Figure 1: Structure and expression of Elfn1. ( a ) Domain structure of Elfn1. LRR, leucine rich repeat; CT, C-terminal domain; FNIII, fibronectin type-III domain; TM, transmembrane domain. ( b ) Subcellular distribution of Elfn1 in the mouse brain. H, homogenates; S1, postnuclear supernatant; P1, nuclear pellet; S2, supernatant after P2 precipitation; P2, crude synaptosomes; S3, cytosol; P3, light membrane; LP1, crude synaptosomal membranes; LP2, synaptic vesicle-enriched fraction; SPM, synaptosomal plasma membranes. ( c , d ) Developmental expression patterns ( c ) and regional distribution ( d ) of Elfn1 protein in mouse brain as analysed by IB. P, postnatal day; W, weeks. ob, olfactory bulb; cc, cerebral cortex; hp, hippocampus; st-gp, striatum and globus pallidus; th, thalamus; ht, hypothalamus; mb, midbrain; po, pons; cb, cerebellum; mo, medulla oblongata; sc, spinal cord. Equal amounts of protein were loaded. ( e ) Immunofluorescence staining of Elfn1 in a frozen sagittal section of adult mouse brain. cc, cerebral cortex; hpf, hippocampal formation; mfb, magnocellular basal forebrain; db, diagonal band; sn, substantia nigra. The picture at right is a magnified view of the hippocampal formation in the picture at left. SUB, subiculum; SP, stratum pyramidale; SR, stratum radiatum; SLM, stratum lacunosum moleculare; SM, stratum moleculare; H, hilus. Scale bar, left, 5 mm. ( f – i ) Double immunofluorescence staining of vibratome coronal sections through the dorsal hp from 4-month-old WT mouse brain with anti-Elfn1 (red) and anti-somatostatin ( f , green, SOM) or anti-PV ( g , green). Scale bars, 100 μm. ( h ) Percentage of double-labelled neurons as a proportion of total Elfn1-positive neurons in the respective layers. ( i ) Percentage of double-labelled neurons as a proportion of the total number of cells immunopositive for SOM or PV. Data were obtained from one hemicoronal section per animal ( n =3 mice). Mean values±s.e.m. are shown. ( j ) Double immunofluorescence staining of the hippocampal CA1 and DG regions. Vibratome coronal sections from 4-month-old WT mouse brain were stained with anti-Elfn1 (magenta) and anti-mGluR1a (green). Images at bottom are magnified images of the boxed regions in the upper image. Closed arrowheads and arrows, Elfn1+ and PV+ soma; open arrowheads, Elfn1+ and PV− soma. Scale bars, 20 μm for upper images and 10 μm for bottom images. Full size image To visualize its protein distribution, we generated an anti-Elfn1 C terminus antibody that does not cross-react with Elfn2, which is another Elfn family protein ( Supplementary Fig. 1a ), and performed immunoblot (IB) ( Fig. 1b−d ) and immunofluorescence staining ( Fig. 1e–g,j and Supplementary Fig. 1b ). A subcellular fractionation analysis revealed that Elfn1 protein was highly enriched in the P2 membrane fraction (which contains myelin, synaptosomes and mitochondria); it was also recovered in the synaptosomal (LP1), synaptosomal plasma membrane (SPM) and postsynaptic density (PSD) fractions, but not in the synaptic vesicle-enriched fraction (LP2) ( Fig. 1b ). These results were consistent with a previous study indicating that Elfn1 localizes mostly to excitatory postsynaptic sites [21] . In the mouse whole brain lysate, Elfn1 was weakly detected during the first week after birth, and strongly detected during 2 to 8 weeks after birth ( Fig. 1c ). In adult brain, Elfn1 was strongly detected in the cerebral cortex, hp, habenular nuclei, septum, diagonal bands, anterior amygdaloid area, globus pallidus and medial forebrain bundles and moderately in the substantial nigra, ventral tegmental nucleus and interpeduncular nuclei ( Fig. 1d,e and Supplementary Fig. 1b ), which is largely consistent with the distribution of Elfn1 mRNA [20] , [22] . In the hp, strong Elfn1 immunoreactivity was detected in the stratum oriens (SO) of the CA1 region, strata oriens and lacunosum of the CA3 region and hilus of the DG ( Fig. 1e ). Elfn1 expression occurs in SOM-INs) [20] , [21] . In our culture system, 96% of the Elfn1-positive neurons were GAD67-positive ( n =51), whereas 35% of the GAD67-positive cells were Elfn1-positive ( n =140) ( Supplementary Fig. 2a ). More than 85% of the Elfn1-positive neurons were SOM-immunopositive in the CA1, CA3 and DG regions ( Fig. 1f,h ; Supplementary Fig. 1c ). Conversely, nearly all of the SOM-positive neurons were immunopositive for Elfn1 ( Fig. 1i ), demonstrating that Elfn1 and SOM largely coexist in the hippocampal interneurons. In addition, around 20% to 30% of the Elfn1-positive neurons were immunopositive for parvalbumin (PV) ( Fig. 1g,h ), suggesting that some Elfn1-positive cells express both SOM and PV. Hippocampal SOM-INs include OLM and oriens-bistratified cells in the CA1 region and HIPP cells in the DG [7] , [23] . Double labelling with Elfn1 and SOM revealed SOM-positive cells with dense Elfn1 signals in the SO and hilus regions ( Fig. 1f ; Supplementary Fig. 1c ), suggesting that Elfn1 is strongly expressed in OLM and HIPP cells. Because OLM and HIPP cells show abundant expression of mGluR1a [8] , [24] , we performed double staining with mGluR1a and Elfn1. As expected, Elfn1 and mGluR1a signals overlapped in the CA1 and hilus regions ( Fig. 1j ). Some of the dendrites of Elfn1- and mGluR1a-positive interneurons in CA1 and most of the dendrites in the hilus possessed spines ( Fig. 1j ), which is another characteristic feature of OLM and HIPP cells. Elfn1 recruits mGluR7 in trans Because multiple LRR-containing transmembrane proteins possess synaptogenic properties [25] , we first performed a neuron–fibroblast co-culture assay to investigate whether Elfn1 or Elfn2 expressed in non-neural cells could induce presynaptic differentiation when contacting axons of co-cultured neurons. However, unlike neuroligin-1, neither Elfn1 nor Elfn2 showed synapse-inducing activity ( Supplementary Fig. 2b,c ). Considering the restricted localization of Elfn1 in OLM and HIPP interneurons, we then hypothesized that Elfn1 could be involved in the regulation of synaptic proteins specific to OLM and HIPP cells. To examine this, rat hippocampal neurons were transfected 7 days after plating (7 days in vitro ) with vectors expressing green fluorescent protein (GFP) or Elfn1 C-terminally tagged with GFP (Elfn1–GFP). Most transfected cells showed a dense distribution of Elfn1–GFP overlapping with the postsynaptic scaffold protein PSD-95, and some were adjacent to a presynaptic protein, Vglut1 ( Supplementary Fig. 3a ). When we immunostained the transfected cells with anti-mGluR7 and anti-mGluR1a antibodies at DIV9, Elfn1–GFP-expressing cells were decorated by mGluR7-immunopositive puncta but were negative for mGluR1a immunoreactivity ( Fig. 2a ; Supplementary Fig. 3a ). In contrast, mGluR7 signals were scarcely detected in GFP-transfected cells ( Fig. 2a ). Endogenous mGluR7-immunoreactive puncta were observed in the vicinity of the GAD67-, mGluR1a- or Elfn1-positive inhibitory neurons at later stages (DIV17, Fig. 2b ; Supplementary Fig. 3b ; DIV51, Fig. 2c ). At a higher magnification, the mGluR7 signals overlapped with the presynaptic marker Vglut1 and were adjacent to Elfn1-immunoreactive signals ( Fig. 2c ). To examine the induction specificity, we expressed mGluR1a–GFP or Flrt3–GFP, which is known to induce presynaptic differentiation through physical interaction with latrophilin 3, a presynaptic seven-pass transmembrane receptor [26] . However, these proteins did not recruit mGluR7, suggesting that the mGluR7-recruiting ability is specific to Elfn1 ( Fig. 2a ). We next expressed Elfn1, mGluR1a and Flrt3 in HEK293 cells, which do not express mGluR7, and co-cultured them with DIV13 hippocampal neurons ( Fig. 2d,e ). Both Elfn1 and Elfn1–GFP recruited mGluR7, whereas mGluR1a–GFP and Flrt3–GFP did not. These results suggest that Elfn1 can recruit mGluR7 in trans and that Elfn1 is sufficient for mGluR7 recruitment in vitro . Consistent with the absence of synaptogenic activity, most mGluR7-positive puncta induced by Elfn1 were separated from Vglut1 signals ( Fig. 2e ). However, when a synaptogenic molecule (neuroligin 2) was co-expressed, mGluR7 puncta signals overlapped with Vglut1, suggesting that Elfn1 can recruit mGluR7 at both synaptic and non-synaptic sites ( Fig. 2e ; Supplementary Fig. 3c ). 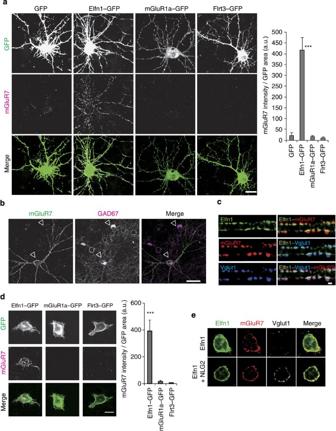Figure 2: Elfn1 recruits mGluR7. (a) Elfn1–GFP can recruit mGluR7 signals. Dissociated hippocampal neurons were transfected with Elfn1–GFP, mGluR1a–GFP, Flrt3–EGFP or EGFP expression constructs at 7 daysin vitro(DIV7). The cells were fixed at DIV9 and immunostained for mGluR7. Scale bar, 20 μm. Graph at right, quantification of mGluR7 intensity normalized to GFP area. a.u. arbitrary unit ***P<0.001, compared with GFP, unpairedt-test.n=24 for GFP,n=23 for Elfn1–GFP,n=24 for mGluR1a–GFP andn=21 for Flrt3–GFP from four independent cultures. (b) Endogenous mGluR7 signals were clustered on inhibitory neurons. Untransfected hippocampal neurons were fixed at DIV17 and double stained for mGluR7 (green) and GAD67 (magenta). Arrowhead indicates the position of the GAD67-positive cell body in each panel. Scale bar, 50 μm. (c) Triple immunolabeling of endogenous Elfn1 (green), mGluR7 (red) and Vglut1 (blue) in untransfected hippocampal neurons at DIV51. mGluR7 signals overlapped with Vglut1 and were adjacent to Elfn1 signals. Scale bar, 1 μm. (d) Elfn1–GFP-transfected HEK293 cells can also recruit mGluR7 signals. Elfn1–GFP transfectants, mGluR1a–GFP transfectants and control Flrt3–GFP transfectants were laid on top of DIV13 hippocampal neurons. Scale bar, 20 μm. The mGluR7 signals in the GFP-positive area were quantified densitometrically (graph at right; a.u.). ***P<0.001, compared with Flrt3–GFP, unpairedt-test.n=7 for Elfn1–GFP,n=15 for mGluR1a–GFP andn=18 for Flrt3–GFP. (e) Elfn1–GFP-expressing HEK293 cells can recruit Vglut1-independent mGluR7 signals while the co-expression of neuroligin 2 (NLG2) can attract mGluR7 signals that partially overlap with Vglut1. Figure 2: Elfn1 recruits mGluR7. ( a ) Elfn1–GFP can recruit mGluR7 signals. Dissociated hippocampal neurons were transfected with Elfn1–GFP, mGluR1a–GFP, Flrt3–EGFP or EGFP expression constructs at 7 days in vitro (DIV7). The cells were fixed at DIV9 and immunostained for mGluR7. Scale bar, 20 μm. Graph at right, quantification of mGluR7 intensity normalized to GFP area. a.u. arbitrary unit *** P <0.001, compared with GFP, unpaired t -test. n =24 for GFP, n =23 for Elfn1–GFP, n =24 for mGluR1a–GFP and n =21 for Flrt3–GFP from four independent cultures. ( b ) Endogenous mGluR7 signals were clustered on inhibitory neurons. Untransfected hippocampal neurons were fixed at DIV17 and double stained for mGluR7 (green) and GAD67 (magenta). Arrowhead indicates the position of the GAD67-positive cell body in each panel. Scale bar, 50 μm. ( c ) Triple immunolabeling of endogenous Elfn1 (green), mGluR7 (red) and Vglut1 (blue) in untransfected hippocampal neurons at DIV51. mGluR7 signals overlapped with Vglut1 and were adjacent to Elfn1 signals. Scale bar, 1 μm. ( d ) Elfn1–GFP-transfected HEK293 cells can also recruit mGluR7 signals. Elfn1–GFP transfectants, mGluR1a–GFP transfectants and control Flrt3–GFP transfectants were laid on top of DIV13 hippocampal neurons. Scale bar, 20 μm. The mGluR7 signals in the GFP-positive area were quantified densitometrically (graph at right; a.u.). *** P <0.001, compared with Flrt3–GFP, unpaired t -test. n =7 for Elfn1–GFP, n =15 for mGluR1a–GFP and n =18 for Flrt3–GFP. ( e ) Elfn1–GFP-expressing HEK293 cells can recruit Vglut1-independent mGluR7 signals while the co-expression of neuroligin 2 (NLG2) can attract mGluR7 signals that partially overlap with Vglut1. Full size image Elfn1 physically interacts with mGluR7 in vivo The above results led us to examine whether Elfn1 associates with mGluR7 in vivo . In immunoprecipitation experiments with mouse brain lysate and an anti-Elfn1 antibody, mGluR7 was co-precipitated with Elfn1 ( Fig. 3a ). Likewise, an anti-mGluR7 antibody co-precipitated Elfn1 ( Fig. 3b ). 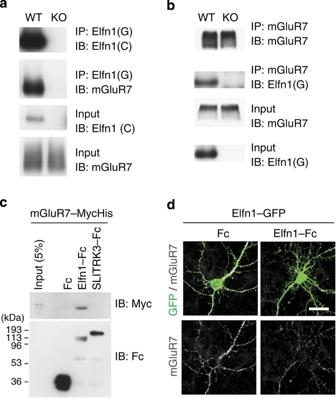Figure 3: Elfn1 binds mGluR7. (a,b) Immunoprecipitation using an anti-Elfn1 antibody (a) and anti-mGluR7 antibody (b). WT and Elfn1 KO brain lysates were subjected to immunoprecipitation (IP) analysis. The co-precipitated mGluR7 (a) and Elfn1 (b) were detected with IB using specific antibodies. G, antibody against the entire cytoplasmic region of Elfn1; C, antibody against the C-terminal 12 residues. (c) Purified Elfn1 ectodomain can bind the mGluR7 ectodomain. Bare Fc protein, Elfn1–Fc protein, SLITRK3–Fc protein and mGluR7–MycHis protein were produced in HEK293 cells and each protein was affinity purified. Fc proteins and mGluR7–MycHis were mixed, and Fc proteins were precipitated with protein G-Sepharose. Precipitated mGluR7–MycHis and Fc proteins were detected with an anti-Myc epitope antibody and anti-Fc antibody, respectively. Blots are representative of at least two biological replicate experiments. (d) Addition of purified Elfn1 ectodomain inhibits the recruitment of mGluR7 in Elfn1–GFP-transfected neurons. Bare Fc or Elfn–Fc proteins were added to the culture media of Elfn1–GFP-transfected neurons at DIV8, which were immunostained for mGluR7 after 36 h. Scale bar, 20 μm. Figure 3: Elfn1 binds mGluR7. ( a , b ) Immunoprecipitation using an anti-Elfn1 antibody ( a ) and anti-mGluR7 antibody ( b ). WT and Elfn1 KO brain lysates were subjected to immunoprecipitation (IP) analysis. The co-precipitated mGluR7 ( a ) and Elfn1 ( b ) were detected with IB using specific antibodies. G, antibody against the entire cytoplasmic region of Elfn1; C, antibody against the C-terminal 12 residues. ( c ) Purified Elfn1 ectodomain can bind the mGluR7 ectodomain. Bare Fc protein, Elfn1–Fc protein, SLITRK3–Fc protein and mGluR7–MycHis protein were produced in HEK293 cells and each protein was affinity purified. Fc proteins and mGluR7–MycHis were mixed, and Fc proteins were precipitated with protein G-Sepharose. Precipitated mGluR7–MycHis and Fc proteins were detected with an anti-Myc epitope antibody and anti-Fc antibody, respectively. Blots are representative of at least two biological replicate experiments. ( d ) Addition of purified Elfn1 ectodomain inhibits the recruitment of mGluR7 in Elfn1–GFP-transfected neurons. Bare Fc or Elfn–Fc proteins were added to the culture media of Elfn1–GFP-transfected neurons at DIV8, which were immunostained for mGluR7 after 36 h. Scale bar, 20 μm. Full size image To address whether the association of Elfn1 and mGluR7 is mediated by their direct physical interaction, we prepared Elfn1 and mGluR7 protein fragments spanning from the amino terminus to their transmembrane domains (ectodomains) as fusion proteins with an immunoglobulin Fc domain and a myc/polyhistidine tag, respectively, to form Elfn1–Fc and mGluR7–MycHis. When the Elfn1–Fc and mGluR7–MycHis were incubated for 1 h at room temperature and the Fc fusion proteins were precipitated with protein G-Sepharose, mGluR7 was co-precipitated ( Fig. 3c ). Co-precipitation was not observed with other reference proteins, either with Fc alone or SLITRK3 ectodomain-Fc (SLITRK3 is an LRR-transmembrane protein known to induce inhibitory synapses by interacting with a receptor protein tyrosine phosphatase, Ptprd [27] ). The addition of Elfn1–Fc to the culture medium of Elfn1–GFP-transfected neurons resulted in 73% lower recruitment of mGluR7 than the addition of Fc alone (Fc, 1.0±0.28; Elfn1–Fc, 0.27±0.07; P =0.019, unpaired t -test, n =12 images, Fig. 3d ). These results indicate that the transinteraction of Elfn1 with mGluR7 is necessary for mGluR7 recruitment. mGluR7 surrounding OLM/HIPP is reduced in Elfn1 KO mice To examine the role of Elfn1 in vivo , we generated Elfn1 KO ( Elfn1 −/− ) mice by homologous recombination in ES cells ( Supplementary Fig. 4a,b ). The absence of Elfn1 protein was confirmed by IB and immunofluorescence staining ( Supplementary Fig. 4c,d ). Specific co-precipitation of mGluR7 or Elfn1 with anti-Elfn1 or mGluR7 was ensured using samples from Elfn1 KO mice ( Fig. 3a,b ). There were no apparent defects in gross brain morphology ( Supplementary Fig. 4e ). To examine whether the synapses on OLM or HIPP interneurons are altered in the hp of Elfn1 KO mice, we compared the localization of mGluR7 and mGluR1a between wild-type (WT) and KO mice ( Fig. 4a–e ). In the hp of WT mice, mGluR7 puncta were densely associated with mGluR1a-positive signals in the outer region of CA1 (OLM in Fig. 4a ) and the hilus of the DG ( Fig. 4a ). By contrast, the association of mGluR7 with mGluR1a-positive signals was rarely observed in KO mice in either region ( Fig. 4a,b ). In the DG, the KO mice had significantly fewer mGluR7-positive spines at both 9 weeks and 4 months ( Fig. 4c ). In other regions, such as the SO and striatum radiatum of CA1, the mGluR7 distribution did not differ between WT and KO mice ( Fig. 4a,b ). 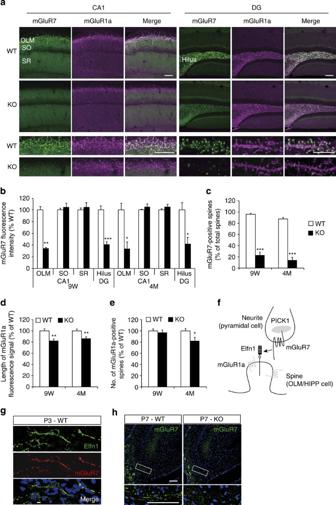Figure 4: mGluR7 distribution is altered in Elfn1 KO hp. (a) Immunostaining for mGluR7 in the CA1 and DG regions. Sections from 4-month-old WT and KO mice were immunostained for mGluR7 (green) and mGluR1 (magenta). The bottom pictures indicate higher magnifications of those at the top. Scale bars, 100 μm (CA1 and upper pictures of DG); 10 μm (bottom pictures of DG). (b) Quantification of the mGluR7-immunopositive signals in hippocampal subregions at 9 weeks (9W) and 4 months (4M). SO, stratum oriens; SR, stratum radiatum. (c) Percentages of mGluR7-positive spines on HIPP cells. For each animal, 5–9 dendrites were analysed. (d,e) The length (d) and number (e) of mGluR1a-positive spine-like structures. (f) Hypothetical positioning of Elfn1, mGluR7 and mGluR1a on pyramidal cell–OLM/HIPP cell excitatory synapses. The model is based on the results shown inFigs. 1. (g) Double staining of Elfn1 and mGluR7 in the prospective stratum oriens from postnatal day 3 (P3) WT mice. Scale bar, 10 μm. (h) mGluR7 signals surrounding the OLM cells are absent in P7 KO mice. Scale bar, 100 μm. (b–e) Mean values±s.e.m. are shown. The values of the WT are set to 100%. *P<0.05, **P<0.01, ***P<0.001, unpairedt-test. (b,c)n=4 (9W);n=3 (4M) mice for each genotype. The measurements from two regions of interest (from right and left hp) were averaged per mouse. (d,e)n=12 sections from four mice for each genotype (9W);n=12 (WT), 11 (KO) sections from three mice for each genotype (4M). Figure 4: mGluR7 distribution is altered in Elfn1 KO hp. ( a ) Immunostaining for mGluR7 in the CA1 and DG regions. Sections from 4-month-old WT and KO mice were immunostained for mGluR7 (green) and mGluR1 (magenta). The bottom pictures indicate higher magnifications of those at the top. Scale bars, 100 μm (CA1 and upper pictures of DG); 10 μm (bottom pictures of DG). ( b ) Quantification of the mGluR7-immunopositive signals in hippocampal subregions at 9 weeks (9W) and 4 months (4M). SO, stratum oriens; SR, stratum radiatum. ( c ) Percentages of mGluR7-positive spines on HIPP cells. For each animal, 5–9 dendrites were analysed. ( d , e ) The length ( d ) and number ( e ) of mGluR1a-positive spine-like structures. ( f ) Hypothetical positioning of Elfn1, mGluR7 and mGluR1a on pyramidal cell–OLM/HIPP cell excitatory synapses. The model is based on the results shown in Figs. 1 . ( g ) Double staining of Elfn1 and mGluR7 in the prospective stratum oriens from postnatal day 3 (P3) WT mice. Scale bar, 10 μm. ( h ) mGluR7 signals surrounding the OLM cells are absent in P7 KO mice. Scale bar, 100 μm. ( b – e ) Mean values±s.e.m. are shown. The values of the WT are set to 100%. * P <0.05, ** P <0.01, *** P <0.001, unpaired t -test. ( b , c ) n =4 (9W); n =3 (4M) mice for each genotype. The measurements from two regions of interest (from right and left hp) were averaged per mouse. ( d , e ) n =12 sections from four mice for each genotype (9W); n =12 (WT), 11 (KO) sections from three mice for each genotype (4M). Full size image Total mGluR1a levels did not differ between WT and KO mice ( Supplementary Fig. 4f,g ). In terms of adjacent Vglut1 signal levels, the mGluR1a-positive neurons in the SO or in hippocampal dissociated culture did not show clear genotype-dependent differences ( Supplementary Fig. 5 ). We further investigated mGluR1a localization within the dendritic spines of WT and KO DG ( Fig. 4d,e ). In 9-week-old mice, the density of mGluR1a-positive spines in the DG hilus did not differ between WT and KO mice ( Fig. 4e ). However, at 4 months of age, KO mice showed a small but significant decrease in spine density ( Fig. 4e ), and the mGluR1a-positive signals within the spines were of shorter length in both 9-week-old and 4-month-old KO mice ( Fig. 4d ). These results indicate that Elfn1 deficiency does not clearly influence synapse formation itself. Taken together with the in vitro experiments, the analysis of Elfn1 KO mice corroborated the role of Elfn1 as a transregulator in recruiting mGluR7 ( Fig. 4f ). We also examined the distribution of Elfn1 and mGluR7 proteins in younger mice. Both Elfn1- and mGluR7-positive signals were detected in partially overlapping regions of WT hippocampi at embryonic day (E) 16, postnatal day 0, P3 and P7 ( Supplementary Fig. 6 ; Fig. 4g,h ). At P3, there were strongly Elfn1-positive and mGluR7-positive signals at the prospective SO layer in WT mice ( Supplementary Fig. 6 ; Fig. 4g ). Double labelling revealed that the two signals were partially overlapping ( Fig. 4g ). At P7, the corresponding mGluR7 signal was detected in WT but not in KO mice ( Fig. 4h ). These results indicate that Elfn1 is required for the recruitment of mGluR7 starting in the early postnatal period. Presynaptic form of plasticity is impaired in KO synapses A previous study revealed that viral vector-mediated Elfn1 knockdown alters the presynaptic form of short-term plasticity of CA1 pyramidal neuron–OLM synapses [21] . To clarify the role of Elfn1 in presynaptic functions in vivo , we recorded excitatory postsynaptic currents (EPSCs) from OLM ( Fig. 5a ) and pyramidal neurons in WT and KO mice and studied the presynaptic form of plasticity. A brief burst stimulation of afferents from CA1 pyramidal neurons induced large short-term facilitation at excitatory synapses onto OLM neurons in WT mice ( Fig. 5b ; n =9 from three mice). By contrast, synapses in KO mice did not show facilitation, and the third, fourth and fifth EPSCs were even depressed ( Fig. 5b ; n =12 from two mice; 10 Hz, second EPSC, P =0.0054, third, P =0.0050, fouth, P =0.0020, fifth, P =0.0023; 20 Hz, second, P =0.031, thirdrd, P =0.014, fourth, P =0.019, fifth, P =0.014, unpaired t -test), suggesting that deleting Elfn1 elevates release probability and impairs short-term plasticity at excitatory synapses onto OLM neurons. In contrast, short-term plasticity of synaptic inputs to pyramidal neurons, used as a reference, was comparable between WT and KO mice ( Fig. 5c,d ; WT, n =15 from two mice; KO, n =13 from two mice), indicating that Elfn1 selectively regulates short-term plasticity at synapses onto OLM neurons. We also investigated long-term potentiation (LTP) at CA1 pyramidal neuron–OLM synapses, which has been reported to be expressed presynaptically [28] . Theta burst stimulation (TBS, see Methods) at −70 mV induced robust LTP of excitatory postsynaptic potentials (EPSPs) in WT mice; however, LTP was much smaller, and long-term depression was even induced by TBS in some OLM neurons in KO mice ( Fig. 5e ; WT, 402.5%±78.8% of baseline 40 min after TBS, n =11 from 10 mice; KO, 116.1%±16.6%, n =10 from 7 mice; P =0.0045; unpaired t -test). To assess the site of expression of this plasticity, we analysed the CV (coefficient of variation , a ratio of s.d. to mean) of EPSPs before and 40 min after TBS [29] . The normalized CV −2 of EPSPs after TBS was higher than the normalized mean EPSP amplitude after TBS in OLM neurons in which LTP was induced, and lower than the normalized means in neurons in which long-term depression was induced ( Fig. 5f ), suggesting that long-term changes induced in OLM neurons were presynaptically expressed. Thus, Elfn1 reduces release probability at pyramidal neuron–OLM neuron synapses while preserving the presynaptic form of LTP and short-term facilitation. 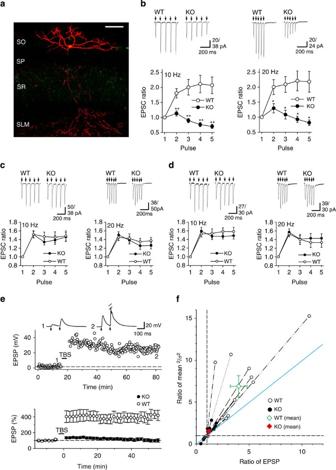Figure 5: Elfn1 preserves short-term facilitation and presynaptic LTP at excitatory synapses onto OLM interneurons. (a) Image of biocytin-filled OLM neuron from WT mouse. The OLM neuron possessed somatostatin in the soma. Green, somatostatin; Red, biocytin; SO, stratum oriens; SP, stratum pyramidale; SR, stratum radiatum; SLM, stratum lacunosum moleculare; scale bar, 100 μm. (b) Short-term facilitation of excitatory synaptic transmission in OLM neurons induced by five successive pulses at 10 Hz (left) and 20 Hz (right) (WT,n=9 from three mice; KOn=12 from two mice). *P<0.05, **P<0.01, unpairedt-test. (c,d) Short-term facilitation at synapses onto CA1 pyramidal neurons in stratum oriens (c) and stratum radiatum (d) (WT,n=15 from two mice; KO,n=13 from two mice). (e) Example of LTP in an OLM neuron from a WT mouse (upper) and summary of LTP in OLM neurons (lower). LTP shown in the upper panel was associated with a decrease in the paired-pulse ratio (insets). An action potential induced by the second pulse in EPSP trace 2 is truncated. (f) Normalized plots of CV−2(ratio of mean2/σ2) versus normalized amplitude of EPSPs before and 40 min after LTP induction (WT,n=11 from 10 mice; KO,n=10 from 7 mice). Suppose that each synapse has a release probability ofpwith a quantal size ofqand that the number of activated synapses isN. Then the amplitude of evoked EPSCs is Npq, and CV−2is equal to Np/(1−p). Ifpincreases after LTP induction, the CV−2plot should be above the diagonal line (blue). Ifpdecreases after long-term depression induction, the CV−2plot should be below the diagonal line. Mean values±s.e.m. are shown. Figure 5: Elfn1 preserves short-term facilitation and presynaptic LTP at excitatory synapses onto OLM interneurons. ( a ) Image of biocytin-filled OLM neuron from WT mouse. The OLM neuron possessed somatostatin in the soma. Green, somatostatin; Red, biocytin; SO, stratum oriens; SP, stratum pyramidale; SR, stratum radiatum; SLM, stratum lacunosum moleculare; scale bar, 100 μm. ( b ) Short-term facilitation of excitatory synaptic transmission in OLM neurons induced by five successive pulses at 10 Hz (left) and 20 Hz (right) (WT, n =9 from three mice; KO n =12 from two mice). * P <0.05, ** P <0.01, unpaired t -test. ( c , d ) Short-term facilitation at synapses onto CA1 pyramidal neurons in stratum oriens ( c ) and stratum radiatum ( d ) (WT, n =15 from two mice; KO, n =13 from two mice). ( e ) Example of LTP in an OLM neuron from a WT mouse (upper) and summary of LTP in OLM neurons (lower). LTP shown in the upper panel was associated with a decrease in the paired-pulse ratio (insets). An action potential induced by the second pulse in EPSP trace 2 is truncated. ( f ) Normalized plots of CV −2 (ratio of mean 2 /σ 2 ) versus normalized amplitude of EPSPs before and 40 min after LTP induction (WT, n =11 from 10 mice; KO, n =10 from 7 mice). Suppose that each synapse has a release probability of p with a quantal size of q and that the number of activated synapses is N . Then the amplitude of evoked EPSCs is Npq, and CV −2 is equal to Np/(1− p ). If p increases after LTP induction, the CV −2 plot should be above the diagonal line (blue). If p decreases after long-term depression induction, the CV −2 plot should be below the diagonal line. Mean values±s.e.m. are shown. Full size image Sensory-triggered seizures in Elfn1 KO mice To investigate higher brain function abnormalities caused by Elfn1 deficiency, we investigated the Elfn1 KO mice at an individual level. Elfn1 KO mice were born at the expected Mendelian ratios (WT, 26.6%; heterozygote, 47.2%; KO, 26.2%; n =778) and the mutation was not lethal. There were no body weight differences at 6 months of age (WT, 33.2±1.2 g, n =7; KO, 33.4±1.2 g, n =12; male mice). Notably, however, we frequently observed seizure-like behaviours of the adult Elfn1 KO mice during routine handling when changing cages ( Fig. 6a ; Supplementary Movie 1 ). To assess their susceptibility to handling-induced seizures, the mice were left undisturbed for 2 weeks before testing, and on the test day, they were picked up by their tail and immediately placed in a new cage. The mice exhibited behavioural signs such as loss of postural equilibrium, Straub tail (arrow in Fig. 6a ), excessive salivation and tonic convulsions during the 2-min observation period; that is, they showed epileptic phenotypes. Handling-induced seizures were observed beginning at 11 weeks after birth ( Fig. 6b ), and the percentage of affected animals peaked (at about 80%) at 5 months ( Fig. 6b ; Supplementary Table 1 ). The handling-induced seizures were observed in both male and female Elfn1 KO mice, but were never observed in WT or Elfn1 heterozygous littermates ( Supplementary Table 1 ). 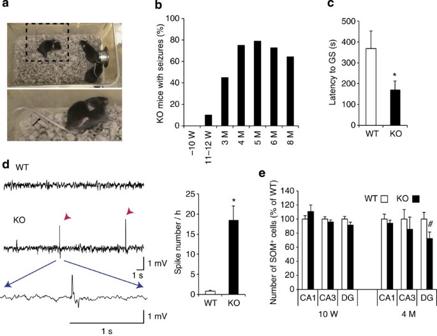Figure 6: Increased seizure susceptibility in Elfn1 KO mice. (a) Handling-induced seizures inElfn1KO mice. Six-month-old KO mice were transferred to a new cage (top panel). Soon after (bottom panel), a mouse (boxed mouse in top panel) showed abnormal movements such as twitching, rigid tail (arrow) and falling down (Supplementary Movie 1). (b) Developmental profile of handling-induced seizures inElfn1KO mice. Percentages of mice that showed seizure-related behaviours were analysed at the indicated stages (numbers are shown inSupplementary Table 1). (c) Increased seizure susceptibility to PTZ administration inElfn1KO mice. Latency to generalized seizures (GS) after intraperitoneal injection of PTZ (50 mg kg−1) was measured in 6-month-old mice. WT,n=7; KO,n=12. Four (57.1%) of 7 WT and 11 (91.7%) of 12 KO mice showed GS within the 600-s observation window; mice without GS were assigned the value of 600 s. Mean values±s.e.m. are shown. *P<0.05, Mann–WhitneyU-test. (d) Representative EEG recordings from 7- to 8-month-old WT and KO mice (left). KO mice showed frequent spike-and-wave-like activity (arrowheads). Right, frequencies of spike waves were measured during the light cycle as the mean number of spikes per hour for WT (n=3) and KO (n=3) mice. *P<0.05, unpairedt-test. (e) SOM-positive cells were counted in the hippocampal CA1, CA3 and DG regions. 10W, WT,n=5; 10W KO,n=6; 4M WT,n=5; 4M KO,n=4 mice.#P=0.08, WT versus KO, unpairedt-test. See alsoSupplementary Fig. S7;Supplementary Table 1andSupplementary Movie. Figure 6: Increased seizure susceptibility in Elfn1 KO mice. ( a ) Handling-induced seizures in Elfn1 KO mice. Six-month-old KO mice were transferred to a new cage (top panel). Soon after (bottom panel), a mouse (boxed mouse in top panel) showed abnormal movements such as twitching, rigid tail (arrow) and falling down ( Supplementary Movie 1 ). ( b ) Developmental profile of handling-induced seizures in Elfn1 KO mice. Percentages of mice that showed seizure-related behaviours were analysed at the indicated stages (numbers are shown in Supplementary Table 1 ). ( c ) Increased seizure susceptibility to PTZ administration in Elfn1 KO mice. Latency to generalized seizures (GS) after intraperitoneal injection of PTZ (50 mg kg −1 ) was measured in 6-month-old mice. WT, n =7; KO, n =12. Four (57.1%) of 7 WT and 11 (91.7%) of 12 KO mice showed GS within the 600-s observation window; mice without GS were assigned the value of 600 s. Mean values±s.e.m. are shown. * P <0.05, Mann–Whitney U -test. ( d ) Representative EEG recordings from 7- to 8-month-old WT and KO mice (left). KO mice showed frequent spike-and-wave-like activity (arrowheads). Right, frequencies of spike waves were measured during the light cycle as the mean number of spikes per hour for WT ( n =3) and KO ( n =3) mice. * P <0.05, unpaired t -test. ( e ) SOM-positive cells were counted in the hippocampal CA1, CA3 and DG regions. 10W, WT, n =5; 10W KO, n =6; 4M WT, n =5; 4M KO, n =4 mice. # P =0.08, WT versus KO, unpaired t -test. See also Supplementary Fig. S7 ; Supplementary Table 1 and Supplementary Movie . Full size image To further evaluate the seizure-prone phenotypes of Elfn1 KO mice, seizure susceptibility was examined by using pentylenetetrazole (PTZ, a GABA A receptor antagonist) as a convulsant. At 6 months, 4 (57%) of 7 WT and 11 (92%) of 12 KO mice showed generalized seizures within 600 s after an intraperitoneal injection of PTZ (50 mg kg −1 ). The latency to generalized seizure was significantly shorter in Elfn1 KO mice than in WT mice ( Fig. 6c ). Epileptic seizures in humans are associated with excessive or abnormally synchronous neuronal discharges. To examine this in the KO mice, we recorded electroencephalogram (EEG) activity from WT and KO mice ( n =3 for each genotype). Five days of monitoring revealed the presence of frequent sharp waves in all three Elfn1 KO mice subjected to the EEG experiment ( Fig. 6d ). These irregular spikes were rarely seen in WT mice ( Fig. 6d ). Spectral analyses of the activity except for sharp waves showed no significant differences between WT and KO mice ( Supplementary Fig. 7a ). SOM-positive hilar neurons are specifically vulnerable to cell death in models of experimental epilepsy [13] . We therefore examined the numbers of interneurons in hippocampal subregions. As expected, the number of SOM-positive hilar interneurons was numerically, although not statistically, reduced in Elfn1 KO mice ( P =0.08) at 4 months but not at 10 weeks, before the onset of seizure ( Fig. 6e ). In contrast, the numbers of PV-positive interneurons in the DG were unchanged at both ages ( Supplementary Fig. 7b ). The tendency of selective loss of hilar SOM-INs is consistent with the seizure-prone phenotypes of Elfn1 KO mice. Collectively, these results revealed sensory-triggered seizures as a cardinal feature of Elfn1 KO mice. Behavioural abnormalities in Elfn1 KO mice In addition to the seizure-prone phenotypes, we observed hyperactivity and impulsivity-related behavioural abnormalities in Elfn1 KO mice. In humans, ADHD is known as a neurodevelopmental disorder characterized by hyperactivity, impulsivity and inattention. In home cages, Elfn1 KO mice showed higher activity than WT mice mainly in the dark phase ( Fig. 7a ). Hyperactive behaviours were observed in several behavioural tasks. In the forced swimming test, the immobility time was reduced ( P =0.0032, Fig. 7b ). In the light–dark box transition test, the total distance travelled and total number of transitions were significantly larger in Elfn1 KO mice than in WT mice ( P =0.00013 and P =0.00055, respectively; Fig. 7c ). Increased total distance travelled was also seen in the elevated plus maze and hole board tests ( Fig. 7d,e ). In the elevated plus maze test, KO mice spent significantly longer time in the open arms ( P =0.0019) and showed more entries into the open arms ( P =0.0019) ( Fig. 7d ), behaviours that are typically regarded as indicative of reduced anxiety. However, this may reflect increased impulsivity rather than reduced anxiety, because there were no signs of reduced anxiety in the light–dark box test ( Fig. 7c , no significant differences in the time spent between the light box and dark box) or in the open field test (no difference in the time spent in the centre area, Supplementary Fig. 8a ). 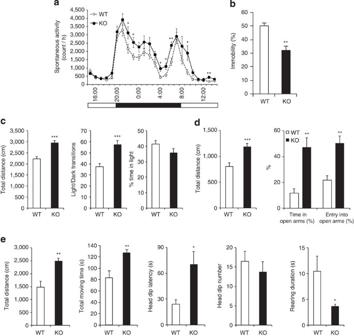Figure 7: ADHD-like behaviours in Elfn1 KO mice. (a–e) Adult WT and Elfn1 KO mice (4–5-month-old,n=10 for each genotype) were used for the behavioural tests. Data shown are means±s.e.m. (a) Spontaneous activity in the homecage. Values are presented as mean±s.e.m. of the activity count per hour. Horizontal bar below the graph indicates the light–dark cycle (black, dark phase; white, light phase). (b) Forced swimming test. Immobility is indicated as a percentage of the 10-min observation period. (c) Light–dark transition test. Total travelled distance, number of transitions from light to dark or from dark to light compartments and percentage of time spent in the light compartment were measured in the test apparatus. (d) Elevated plus maze test. Total travelled distance, percentage of time spent in the open arms in the 5-min observation period and entry into open arms as a percentage of the total entries into the arms were measured. (e) Hole board test. Total travelled distance, total moving time, latency to the first head dip, number of head dips and rearing duration were measured over the 5-min observation period. (a–e) *P<0.05, **P<0.01, ***P<0.001, unpairedt-test for parameters other than percentage, Mann–WhitneyU-test for percentage data. See alsoSupplementary Fig. 8. Figure 7: ADHD-like behaviours in Elfn1 KO mice. ( a – e ) Adult WT and Elfn1 KO mice (4–5-month-old, n =10 for each genotype) were used for the behavioural tests. Data shown are means±s.e.m. ( a ) Spontaneous activity in the homecage. Values are presented as mean±s.e.m. of the activity count per hour. Horizontal bar below the graph indicates the light–dark cycle (black, dark phase; white, light phase). ( b ) Forced swimming test. Immobility is indicated as a percentage of the 10-min observation period. ( c ) Light–dark transition test. Total travelled distance, number of transitions from light to dark or from dark to light compartments and percentage of time spent in the light compartment were measured in the test apparatus. ( d ) Elevated plus maze test. Total travelled distance, percentage of time spent in the open arms in the 5-min observation period and entry into open arms as a percentage of the total entries into the arms were measured. ( e ) Hole board test. Total travelled distance, total moving time, latency to the first head dip, number of head dips and rearing duration were measured over the 5-min observation period. ( a – e ) * P <0.05, ** P <0.01, *** P <0.001, unpaired t -test for parameters other than percentage, Mann–Whitney U -test for percentage data. See also Supplementary Fig. 8 . Full size image Elfn1 KO mice also showed intriguing behavioral abnormalities in the hole board test. In this test, mice were placed in an open-field-like box with four floor holes, and their exploration of the holes was analysed. Latencies to dipping their heads into all holes was prolonged in Elfn1 KO mice ( P =0.014), whereas the total number of head dips (probably reflecting investigation) did not differ between the genotypes ( Fig. 7e ). In addition, the total time of rearing, a posture indicating alertness, was lower in Elfn1 KO mice ( P =0.047, Fig. 7e ). These results implicate the altered cognition of the experimental environment in Elfn1 KO mice. Lack of Elfn1 had no effect on sensory–motor gating function as assessed by the prepulse inhibition test, or pain sensitivity as evaluated with the hot plate and tail flick tests ( Supplementary Fig. 8b–d ). Mutations of ELFN1 in patients with neurological disorders Having observed the neurological phenotypes of Elfn1 KO mice, we performed re-sequence analysis of the ELFN1 complete open reading frame in subjects who were clinically diagnosed with epilepsies (total n =184, 119 idiopathic generalized epilepsy and 65 symptomatic epilepsy) or autism spectrum disorder (ASD; n =316), some of whom had comorbid attention deficit hyperactivity disorder (ADHD), and healthy control subjects ( n =311) ( Supplementary Table 2 ). All of the patients and control individuals examined in this study were Japanese, a population that has been reported to have little or negligible stratification [30] . We identified four novel heterozygous missense mutations (c.1442C>T, c.1948C>T, c.2032G>A and c.2071C>T) resulting in the amino-acid substitutions p.Ala481Val, p.Arg650Cys, p.Asp678Asn and p.Arg691Trp, respectively; these were detected only in patients ( Table 1 ), and not in mentally healthy subjects ( n =2480). The mutations were in four patients from different families who were diagnosed with Asperger syndrome (A481V), Asperger syndrome/ADHD (R650C), childhood absence epilepsy/ADHD (D678N) and juvenile myoclonic epilepsy (R691W) ( Table 1 ). However, A481V was not found in an affected sibling, suggesting that this mutation does not have 100% penetrance. Table 1 ELFN1 mutations and clinical phenotypes. Full size table Interestingly, R650C, D678N and R691W were clustered in the cytoplasmic region ( Fig. 8a ) and were scored as possibly (D678N) or probably (R650C, R691W) damaging by the PolyPhen-2 algorithm [31] . We therefore set out to perform functional evaluation of these three mutants, although we could not detect statistically significant differences in the overall or any single variant allele frequencies between cases and controls. When we transfected constructs expressing the human WT ELFN1 or the three ELFN1 variants into hippocampal neurons, R650C, D678N and R691W recruited significantly lower amounts of mGluR7 signal than WT ELFN1 ( Fig. 8b,c ). Other missense mutations (R496G and R744G) did not show any significant impairment in recruiting activities. These results indicate that the R650C, D678N and R691W mutations are all functionally defective in terms of mGluR7-recruiting activities. In addition, the ELFN1-immunopositive signals were reduced for the R650C and D678N variants ( Fig. 8d,e ). Collectively, these results suggest that the identified ELFN1 variants could have a pathological role in a subset of patients with neurological disorders. 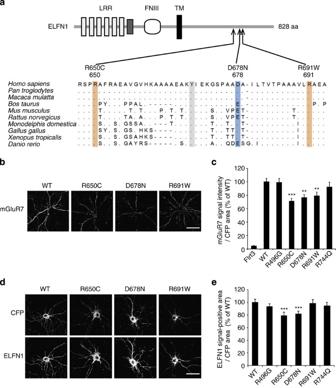Figure 8:ELFN1missense mutations identified in patients with epilepsy or ADHD. (a) R650C, D678N and R691W were missense SNPs found only in the patient cohorts. The three mutations were clustered in the C-terminal region ofELFN1. Amino-acid sequences of the corresponding regions were aligned from various vertebrate species. Orange, absolutely conserved position (R650, R691); blue, conservative amino-acid position (D678), grey, an absolutely conserved tyrosine in the sequences. (b) Representative immunostaining images for mGluR7 in the hippocampal neurons expressing WTELFN1,ELFN1R650C,ELFN1D678N andELFN1R691W. The hippocampal neurons were transfected with pCAG-ires-ECFP-based plasmid vectors. Scale bar, 50 μm. (c) Quantitative analysis of mGluR7 signals as a percentage of the CFP-positive area. The densitometrically measured signal intensity is shown in a.u.n=82 neurons for Flrt3,n=131 for WT,n=77 for R496G,n=105 for R650C,n=85 for D678N,n=79 for R691W andn=72 for R744Q from three independent experiments. (d) Representative immunostaining images for ELFN1 in the same transfectants as shown in (b). Scale bar, 50 μm. (e) Quantitative analysis of Elfn1 signals overlapped with CFP signals.n=51 neurons for WT,n=52 for R496G,n=47 for R650C,n=50 for D678N,n=50 for R691W andn=49 for R744Q from four independent experiments. Mean values±s.e.m. are shown. **P<0.01, ***P<0.001, unpairedt-test. See alsoSupplementary Table 2. Figure 8: ELFN1 missense mutations identified in patients with epilepsy or ADHD. ( a ) R650C, D678N and R691W were missense SNPs found only in the patient cohorts. The three mutations were clustered in the C-terminal region of ELFN1 . Amino-acid sequences of the corresponding regions were aligned from various vertebrate species. Orange, absolutely conserved position (R650, R691); blue, conservative amino-acid position (D678), grey, an absolutely conserved tyrosine in the sequences. ( b ) Representative immunostaining images for mGluR7 in the hippocampal neurons expressing WT ELFN1 , ELFN1 R650C, ELFN1 D678N and ELFN1 R691W. The hippocampal neurons were transfected with pCAG-ires-ECFP-based plasmid vectors. Scale bar, 50 μm. ( c ) Quantitative analysis of mGluR7 signals as a percentage of the CFP-positive area. The densitometrically measured signal intensity is shown in a.u. n =82 neurons for Flrt3, n =131 for WT, n =77 for R496G, n =105 for R650C, n =85 for D678N, n =79 for R691W and n =72 for R744Q from three independent experiments. ( d ) Representative immunostaining images for ELFN1 in the same transfectants as shown in ( b ). Scale bar, 50 μm. ( e ) Quantitative analysis of Elfn1 signals overlapped with CFP signals. n =51 neurons for WT, n =52 for R496G, n =47 for R650C, n =50 for D678N, n =50 for R691W and n =49 for R744Q from four independent experiments. Mean values±s.e.m. are shown. ** P <0.01, *** P <0.001, unpaired t -test. See also Supplementary Table 2 . Full size image We have demonstrated a novel molecular function of Elfn1 in binding to mGluR7 and recruiting presynaptic mGluR7-containing processes to Elfn1-expressing SOM-INs. The importance of the interaction was substantiated by the demonstration of their binding at the synapse level and by manifold phenotypic data from Elfn1 KO mice. mGluR7 was originally identified as a seven-membrane-spanning G-protein-coupled receptor [32] belonging to the Group III (mGluR4, mGluR6, mGluR7, mGluR8) metabotropic glutamate receptor family, whose members are known to regulate synaptic transmission [33] . mGluR7 is broadly expressed in the central nervous system, with strong expression in CA1, CA3 and the granule cells of the DG [34] , [35] . In the hp, mGluR7 proteins are detected presynaptically [36] in a target cell (OLM)-specific manner [10] , [11] . Furthermore, the distribution of mGluR7 is dynamically controlled. mGluR7 is internalized in response to activation by the glutamate agonists L-AP4 [37] and AMN082 [38] , and the dynamics of mGluR7 have been proposed as a core mechanism that affects the plasticity of hippocampal mossy fibre–CA3 stratum lucidum interneurons [37] . However, to our knowledge, there have been no reports of mGluR7 regulators other than glutamate and its synthetic agonists, such as L-AP4 and AMN082, which can bind the N-terminal ectodomain. Elfn1 is thus the first identified endogenous transregulator of mGluR7. The seizure-prone phenotype of the Elfn1 KO mice is remarkably similar to that of mGluR7 KO mice, which show late-onset sensory stimulus-induced seizures after cage transfer (beginning at 10 weeks old, and not occurring at 6 to 8 weeks old) [14] . Furthermore, increased PTZ-induced seizure susceptibility has also been observed in mGluR7 KO mice [14] . These phenotypic similarities, together with the molecular and functional linkage between Elfn1 and mGluR7, can explain the pathophysiological basis of the seizure-prone phenotypes shared by Elfn1 and mGluR7 KO mice. Considering the essential role of the mGluR7–PICK1 interaction in suppressing seizure susceptibility [15] , [16] as well as in presynaptic clustering [18] and surface expression [39] of mGluR7, the impaired mGluR7 distribution may be responsible for the seizure-prone phenotype of Elfn1 KO mice. Missense mutations of ELFN1 identified in patients with epilepsy, ADHD, and/or ASD were located in the intracellular region and did not substantially affect protein stability. However, the distribution of mGluR7 was slightly but significantly reduced in our in vitro experiments, suggesting an as-yet-unidentified postsynaptic mechanism that may stabilize the Elfn1–mGluR7 interaction. A brief train of afferent stimulation induced short-term depression rather than short-term facilitation at CA1 pyramidal neuron–OLM neuron synapses in Elfn1 KO mice ( Fig. 5b ), suggesting that Elfn1 reduces release probability [21] . We speculate that a decrease in mGluR7 at these synapses elevated the release probability in KO mice, because group III mGluRs reduce transmitter release [40] . We also found that LTP at pyramidal neuron–OLM neuron synapses was impaired in Elfn1 KO mice ( Fig. 5e ). LTP at excitatory synapses on interneurons was associated with an increase in release probability at presynaptic sites ( Fig. 5f ), and LTP was possibly occluded by the original higher release probability in KO mice. In addition, LTP in OLM interneurons also depends on postsynaptic calcium-permeable AMPA receptors [28] ; therefore, we also hypothesize that the Elfn1–mGluR7 interaction may have a role in coordinating the retrograde regulation of presynaptic terminals by OLM interneurons. Because neither we nor Sylwestrak et al . [21] observed typical synapse formation-inducing activity, Elfn1 is probably not a conventional synaptic organizer but rather regulates specific synaptic properties. Although the question of how PICK1 and other mGluR7-binding partners mediate the suppression of release probability remains unresolved, further analysis of the molecular function of Elfn1 may enable us to decipher the mechanisms underlying the diversity of synaptic function. There are two major questions raised by the current study. First, why does the seizure-prone phenotype appear in the later stage of development in both Elfn1 and mGluR7 KO mice? Given that a reduction of Elfn1 can enhance the presynaptic release probability at pyramidal–OLM synapses, reduced Elfn1 may lead to disorganized dendritic inhibition by OLM interneurons, further affecting network excitability. This sustained higher synaptic activity may result in the loss of interneurons, which is relevant to the mild decrease of SOM-INs after the onset of seizures in Elfn1 KO mice ( Fig. 6e ) and to GABAergic dysfunction in mGluR7 KO mice as previously shown by decreased mRNA levels of hippocampal GAD65 and GAD67 in 12- to 16-week-old mice [41] . The dysfunction of SOM-INs has been proposed as a cause of both experimental and human temporal lobe epilepsy (reviewed in ref. 42 ). Seizures induce the loss of SOM-INs in the DG [12] , [43] , [44] , and there is an electrophysiologically detectable reduction in GABA release [13] , [45] . Seizure models based on Elfn1–mGluR7 dysfunction may shed new light on the role of SOM-INs in epileptogenesis. Because SOM has an inhibitory effect on the hp, and the SOM system has been suggested as a potential target for antiepileptic drugs [42] , further clarification of Elfn1–mGluR7 function would be beneficial for both treating epilepsies and understanding their pathophysiological mechanisms. The second question is how ELFN1 mutations are involved in the pathogenesis of neurological disorders. Epilepsy is complicated by ADHD in 20–31.5% of cases, and ADHD is associated with high rates of electroencephalographic abnormalities [46] , [47] , suggesting that epilepsy and ADHD share a common pathophysiology in a subset of patients. The comorbidity may be partly due to genetic factors that are involved in both epilepsy and ADHD pathogenesis. In this regard, ELFN1 appears to be a candidate gene. Further clarification of its domain functions, in particular the function of the domain in which clustered missense mutations are detected (aa 650–691), will be important because structural changes impaired mGluR7-binding activity. Because this region contains residues that are strongly evolutionarily conserved, our current hypothesis is that some of these regions may interact with signal transducing adaptor proteins. The signalling may affect protein localization, as found for R650C and D678N, or some other unknown function of Elfn1. Since we used a full-KO model of Elfn1, and Elfn1 is expressed not only in the hp but also in the neocortex, subiculum and several other regions, it will be essential to correlate each behavioural abnormality with the responsible neural circuit through conditional gene targeting. In previous studies, GRM7 (mGluR7) has been shown to be associated with neurological disorders such as schizophrenia, hearing impairment and ADHD [48] , [49] , [50] . Although ELFN1 has not been reported as a major genetic factor for any neuropsychiatric disorder, we expect that further genetic investigation will demonstrate its involvement in neurodevelopmental disorders other than epilepsy and ADHD, given the shared genetic architecture among mental disorders that has been revealed in recent studies [51] , [52] . In summary, the current study highlights the novel physiological roles of Elfn1, including its contribution to the synaptic properties of the SOM-INs, which may be relevant to the neurological phenotypes seen with the loss of Elfn1 function. Our results in both the mouse and human suggest that the Elfn1–mGluR7 system constitutes an indispensable core mechanism for tuning the excitability of mammalian brains. Ethics statement All animal experiments were approved by the institutional ethical committees and carried out in accordance with the guidelines for animal experimentation in RIKEN, Nagasaki University Graduate School of Biomedical Sciences, and Gunma University Graduate School of Medicine. Antibodies The following antibodies were purchased from the indicated companies: actin (A2066, Sigma, 1:1,000 dilution for IB), PSD-95 (MA1-045, Thermo Scientific, 1:5,000 dilution for IB; 1:100 dilution for immunocytochemistry), synaptophysin (S5768, Sigma, 1:10,000 dilution for IB; 1:200 for immunocytochemistry), synapsin-I (Millipore, 1:1,000), somatostatin (sc-7819, Santa Cruz, 1:2,500 dilution for immunofluorescence staining of vibratome sections; 1:250 dilution for immunostaining of frozen sections), parvalbumin (P3088, Sigma, 1:5,000 dilution for immunofluorescence staining of vibratome sections; 1:4,000 dilution for immunostaining of frozen sections), gephyrin (mAb7a, Synaptic Systems, 1:250 dilution for immunocytochemistry), GAD67 (MAB5406, Millipore, 1:250 dilution for immunocytochemistry), mGluR7 (07-239, Millipore, 1:2,000 dilution for IB; 1:100 dilution for immunocytochemistry; 1:2,000 dilution for immunofluorescence staining of vibratome sections), mGluR1a (G209-488, BD Pharmingen, 1:1,000 for immunocytochemistry; 1:2,000 dilution for immunofluorescence staining of vibratome sections), GluR5 (N-19, Santa Cruz, 1:1,000 for IB), PICK1 (N-18, Santa Cruz, 1:1,000 for IB), Vglut1 (AB5905, Millipore, 1:400 for immunocytochemistry; 1:500 for immunostaining for frozen section), Myc (9E10, Santa Cruz, 1:500 dilution for IB), HA (12CA5, Roche, 1:500 for IB), Fc (109-035-098, Jackson Immunoresearch, 1:10,000), and GFP (3E6 and chicken polyclonal, Invitrogen, 1:500 dilution for immunocytochemistry). For production of anti-Elfn antibodies, rabbits were immunized with a synthesized C-terminal Elfn1 peptide (aa 817–828), purified Elfn1–GST (glutathione S -transferase) or Elfn2–GST fusion protein by following a standard protocol. cDNA fragments including the C-terminal domains of mouse Elfn1 (aa 635–828) and mouse Elfn2 (aa 545–823) were subcloned into the pGEX-6P2 plasmid (GE Healthcare) for expression of GST fusion proteins in E. coli BL21 (DE3). The GST fusion proteins were purified using glutathione Sepharose 4B (GE Healthcare) and used for immunization. The obtained antisera were purified by affinity chromatography with the peptide used for immunization or GST fusion proteins. Antibodies raised against Elfn1–GST and Elfn2–GST fusion proteins were further passed through an Elfn2–GST fusion protein-conjugated column and an Elfn1–GST fusion protein-conjugated column, respectively. Animals Elfn1 -deficient mice were generated as described previously [53] . Briefly, to construct the Elfn1 targeting vector, overlapping Elfn1 genomic clones were obtained from BACPAC Resources Center at Children’s Hospital Oakland Research Institute (Oakland, CA). The targeting construct contained the 4.5-kb 5′ and 5.9-kb 3′ homology regions, and the 3.5-kb fragment containing the open reading frame of Elfn1 was replaced with the phosphoglycerol kinase (PGK)–neo expression cassette flanked by a loxP sequence. Embryonic stem cells (EmbryoMax Embryonic Stem Cell Line—Strain C57BL/6, Millipore) were electroporated with the targeting construct and selected with G418. Drug-resistant clones were analysed by Southern blotting. Chimeric mice were generated by injection of the targeted embryonic stem cells into BALB/c blastocysts. To excise the PGK–neo cassette, mice with germline transmission were first mated with transgenic mice expressing Cre recombinase in germline cells [53] . Correct excision of the PGK–neo cassette was confirmed by Southern blot. The resulting ( Elfn1 +/− , Cre-transgene) mice were backcrossed once to C57BL/6J mice to remove the Cre-transgenes. Elfn1 +/– heterozygotes were used to generate Elfn1 –/– mice, which are referred to as Elfn1 KO mice in this study. Genotyping was performed by Southern blot or PCR analysis of DNA isolated from tail samples. All experiments used male mice unless otherwise noted. Immunoblotting Regional and developmental specimens and subcellular fractions were prepared and subjected for IB as previously described [53] , [54] , [55] . For preparation of subcellular fractions, whole mouse brain was homogenized in buffered sucrose solution A (320 mM sucrose, 5 mM HEPES-KOH, pH 7.4) and centrifuged at 800 g for 10 min to obtain S1 fraction. S1 fraction was further centrifuged at 10,000 g for 30 min to obtain S2 fraction. S2 fraction was centrifuged at 100,000 g for 1 h to obtain S3 fraction. P2 crude synaptosomal fraction was homogenized in solution A and layered on sucrose gradient (0.85 M, 1.0 M and 1.2 M sucrose containing 5 mM HEPES). After centrifugation at 100,000 g for 2 h in a Beckman SW55Ti rotor, synaptosomal fraction was collected between 1.0 M and 1.2 M sucrose. Synaptosomal fraction was resuspended in buffered sucrose, lysed in 6 mM Tris–HCl (pH 8.0) and agitated at 4 °C for 45 min. LS1 and LP1 fraction was obtained after centrifugation at 32,800 × g for 20 min and LS1 fraction was further centrifuged at 165,000 g for 2 h to obtain LP2 pellet. LP1 pellet was resuspended in solution B (0.16 M sucrose in 6 mM Tris–HCl (pH 8.0) containing 1% Triton X-100 and protease inhibitor cocktail) and agitated at 4 °C for 15 min. After centrifugation at 32,800 g for 20 min, the resultant pellet was resuspended in solution B and layered on sucrose gradient (1.0 M, 1.5 M and 2.0 M sucrose containing 5 mM HEPES). After centrifugation at 201,000 g for 2 h in a Beckman SW55Ti rotor, synaptosomal plasma membrane and crude PSD fractions were collected above the 1.0 M layer of between 1.5 M and 2.0 M layer, respectively. Crude PSD fraction was resupended in modified solution B containing 75 mM KCl and agitated at 4 °C for 15 min. Purified PSD fraction was obtained after centrifugation at 201,000 g for 20 min. Whole or parts of mouse brains from each developmental stage or region were homogenized in RIPA buffer (50 mM Tris–HCl pH 8.0, 150 mM sodium chloride, 1% NP-40, 0.5% sodium deoxycholate, 0.1% SDS, 1 mM EDTA and protease inhibitor cocktail. Protein extracts were separated by SDS–polyacrylamide gel electrophoresis and transferred to polyvinylidene fluoride (Immobilon-P, Millipore) membranes. The membranes were blocked with 5% skim milk in phosphate-buffered saline (PBS) containing 0.1% Tween20 and probed with primary antibodies, followed by incubation with secondary antibodies conjugated to horseradish peroxidase. Blots were developed with ECL Plus reagents (GE Healthcare) and exposed to Hyperfilm ECL (GE Healthcare). Immunostaining for brain sections Mice were anaesthetized and perfused transcardially with 4% paraformaldehyde (PFA) in 0.1 M phosphate buffer (pH 7.4). The brains were removed, postfixed for 3 h at 4 °C and sectioned at a thickness of 50 μm on a vibratome. Free-floating vibratome sections were incubated in blocking solution (PBS containing 10% normal goat serum and 0.1% Triton X-100) overnight, followed by incubation with primary antibodies for 3 days and with Alexa 488- or Alexa 594-conjugated secondary antibodies (Molecular Probes) overnight at 4 °C. To prepare the cryostat sections (12 μm), postfixed brains were cryoprotected in 20% sucrose (wt/vol) in PBS for 48 h at 4 °C, embedded in OCT compound and frozen on dry ice. For immunofluorescence staining, cryostat sections were incubated in blocking solution (PBS containing 10% normal goat serum and 0.1% Triton X-100) for 1 h at room temperature, followed by incubation with primary antibodies overnight at 4 °C and with Alexa 488- or Alexa 594-conjugated secondary antibodies (Molecular Probes) for 1 h at room temperature. For cell counting analyses for SOM- or PV-positive interneurons, cryostat sections were autoclaved in 10 mM citrate buffer, pH 6.0, for 5 min at 105 °C for antigen retrieval (SOM) and incubated in 0.3% H 2 O 2 /methanol for 10 min. After incubation in blocking solution for 1 h at room temperature, sections were incubated with primary antibodies overnight at 4 °C and visualized by using the Vectastain ABC Elite system (Vector Laboratories). Direct labelling of the anti-Elfn1 antibody was carried out by using the Fluorescein labelling kit NH 2 (Dojindo). Immunostaining was performed at least three times with independent mouse brain sections and representative pictures were shown. Primary neuronal cultures and immunostaining Primary neuronal cultures were prepared from the hippocampi of (E) 18/19 Sprague–Dawley rats or (E) 16 mice. Briefly, the hippocampi were dissociated by treatment with trypsin EDTA and gently triturated with a pipette. The dissociated cells were plated onto poly- D -lysine-coated coverslips in Neurobasal medium supplemented with B27 (Invitrogen) and 2 mM L -glutamine. Cultured cells were transfected with Lipofectamine 2000 (Invitrogen) according to the manufacturer’s protocol. The frequency of the GAD67-positive cells in the GFP-positive transfectant was very low (0.3%) in our experimental system. For immunofluorescence staining of synaptic marker proteins, neurons were fixed with 4% PFA/4% sucrose in PBS on ice for 40 min or for 30 min followed by incubation in pre-chilled methanol for 10 min. Neurons were then permeabilized with Triton X-100, blocked with 5% normal goat serum and incubated with the primary and fluorescently labelled secondary antibodies. For mGluR7 staining, neurons were fixed with 100% methanol at −20 °C for 5 min and then incubated with primary and secondary antibodies in 30 mM phosphate buffer pH 7.4 containing 0.2% gelatin, 0.5% Triton X-100 and 0.8 M NaCl. DNA constructs Mouse Elfn1 cDNA was obtained through the FANTOM cDNA resource ( http://fantom.gsc.riken.jp/ ). The open reading frame was PCR amplified and inserted into the pEF1-MycHis plasmid vector (Invitrogen). PCR-generated EGFP sequences that were in-frame with the Elfn1 sequence were inserted at an XbaI site in the C-terminal flanking sequence. To construct the Elfn1–Fc fusion protein expression vector, the PCR-generated Elfn1 ectodomain cDNA fragment was first inserted into the pAP-tag5 vector (GeneHunter). The resultant Elfn1 ectodomain sequence preceded by the immunoglobulin signal peptide sequence was PCR amplified and inserted into the pEF-Fc vector (a gift from Dr Yoshihiro Yoshihara, RIKEN BSI), allowing the target protein to be fused at the C terminus to the Fc region of human IgG1. The WT ELFN1 vector was generated by inserting human ELFN1 protein coding regions PCR amplified from the genomic DNA of a healthy human subject and cloned into the pGEMT easy plasmid vector (Promega). PCR-based site-directed mutagenesis was carried out by using appropriate primers for R650C, D678N and R691W. The resultant NotI fragments containing the entire protein coding region preceded by the Kozak consensus sequence were inserted into pCAG-ires-ECFP vectors in which ECFP was modified to have a GAP43-derived membrane anchor signal sequence. mGluR7 cDNA was PCR cloned by using Mouse 17-day Embryo Marathon-Ready cDNA (Clontech). The cDNA fragment was first inserted into the pAP-tag5 vector, and the intervening alkaline phosphatase sequence was removed by restriction endonuclease digestion, resulting in the mGluR7 ectodomain tagged at the C terminus with MycHis epitopes (pEF-mGluR7ecto-MycHis). The Flrt3 expression vector was constructed by PCR, using a mouse Flrt3 cDNA clone (FANTOM cDNA resource). The human SLITRK3 expression vector will be described elsewhere. The mGluR1aEGFP expression vector was provided by Dr Akihiro Mizutani (Showa Pharmaceutical University). Synapse induction assay Artificial synapse formation assays were performed with HEK293T cells as described [56] . The plasmids used in this experiment are pCMV5-NL1ΔAB EGFP, pCAG-Elfn1-iresEGFP, pCAG-Elfn2-iresEGFP and pCAG-iresEGFP alone. mGluR7-recruiting activity assay HEK293T cells were transfected with pCAG-ires-EGFP-based expression constructs by using TransIT LT1 reagent (Mirus Bio). After 48 h, cells were trypsinized, suspended in Neurobasal/B27 medium and laid onto the hippocampal neurons at DIV13 at a density of 1.5 × 10 4 cells. The co-cultured cells were maintained for 24 h, chilled on ice for 5 min and fixed with 4% PFA, 4% sucrose in PBS at 4 °C for 20 min. After four washes with PBS, the cells were immersed in a blocking buffer (5% normal goat serum, 3% bovine serum albumin, 0.1% Triton X-100 in PBS) and incubated with rabbit anti-mGluR7 and chicken anti-GFP diluted in the blocking buffer overnight at 4 °C. The bound antibodies were detected by Alexa 594-conjugated anti-rabbit IgG and Alexa 488-conjugated anti-chicken IgY (Jackson Immunoresearch). In vitro mGluR7-pull down binding assay The Fc fusion protein was produced in HEK293T cells and affinity purified using protein G-Sepharose. HEK293T cells in a 10-cm dish were transfected with pEF-mGluR7ecto-MycHis. The cells were lysed in 1 ml of a buffer consisting of 0.5% Triton X-100, 150 mM NaCl and 50 mM Tris–HCl pH 7.5 with Complete Protease Inhibitor Cocktail (Roche). After incubation for 20 min at 4 °C with gentle rocking, the lysate was centrifuged at 13,000 g for 20 min at 4 °C. For the binding assay, 50 μl of the supernatant was mixed with 950 μl of a binding buffer (10 mM HEPES, pH 7.4, 2 mM CaCl 2 , 1 mM MgCl 2 and 0.1% Triton X-100) containing 1.5 μg of Fc or Fc fusion proteins, and was incubated for 1 h at 4 °C with gentle agitation. After the binding reaction, the binding mixture was added by ImmunoPure Immobilized Protein G (Pierce), and further incubated for 1 h at 4 °C, followed by brief spinning. The proteins co-precipitated with the Protein G-resin were washed four times with the binding buffer and analysed by IB. Imaging and quantitative immunofluorescence analysis Image acquisition and analysis were performed by investigators blind to the experimental condition. For immunofluorescence experiment, single-plane images were captured using a FV1000 confocal microscope (Olympus) or BIOREVO BZ-9000 (Keyence) with identical settings. For transfected neurons, GFP- or CFP-expressing neurons were randomly chosen and imaged. The intensity values from the thresholded images were obtained using ImageJ software ( http://rsb.info.nih.gov/ij/ ). For quantitative analysis of mGluR7 levels in brain sections, rectangular regions of interest were defined for CA1, SO and SR, and the intensity values from the thresholded images were obtained using ImageJ software. The regions of interest in CA1, OLM and DG hilus were determined from the mGluR1a-positive area. mGluR1a-positive spines were manually counted and normalized to 10-μm dendrite lengths. The length of the mGluR1a-positive structure was defined as the length from the dendrite to the tip of the mGluR1a-positive protrusions. For cell counting analysis of somatostatin- or PV-positive interneurons in the hp, images were acquired with a NanoZoomer slide scanner (Hamamatsu Photonics). Immunoprecipitation The crude synaptosomal (P2) fraction of mouse hippocampi was incubated in co-immunoprecipitation buffer (10 mM Tris–HCl pH 7.5, 150 mM NaCl, 1% Nonidet P-40, 1 mM EDTA) supplemented with protease inhibitor cocktail for 1 h at 4 °C. The lysates were obtained by centrifugation for 30 min at 10,000 g , precleaned with anti-rabbit IgG agarose beads (Sigma), and incubated with 0.5 μg anti-Elfn1 or anti-mGluR7 antibodies. Complexes were isolated using anti-rabbit-IgG agarose beads. Slice electrophysiology Slices were prepared from adult (postnatal week 11–32) Elfn1 KO mice or their WT littermates by using the protective recovery method [57] . Transverse slices were used for recording pyramidal cells and coronal slices were used for recording OLM neurons. Mice were anaesthetized with isoflurane and sodium pentobarbital and transcardially perfused with a room temperature carbogenated (95% O 2 and 5% CO 2 ) protective artificial cerebrospinal fluid (ACSF) containing 92 mM N -methyl- D -glucamine, 2.5 mM KCl, 1.2 mM NaH 2 PO 4 , 30 mM NaHCO 3 , 20 mM HEPES, 25 mM glucose, 5 mM ascorbate, 3 mM sodium pyruvate, 12 mM N -acetyl- L -cysteine, 0.5 mM CaCl 2 and 10 mM MgSO 4 . The mice were then decapitated, the brains were removed and hippocampal slices were cut using a vibrating blade microtome (VT1200S, Leica) at room temperature. When cutting transverse hippocampal slices, the hp was dissected before slicing. The hippocampal slices were recovered in the carbogenated protective ACSF at 32 °C for 12 min and then transferred into a holding chamber containing a room temperature carbogenated incubating ACSF of the following composition: 119 mM NaCl, 2.5 mM KCl, 1 mM NaH 2 PO 4 , 26.2 mM NaHCO 3 , 12.5 mM glucose, 2 mM CaCl 2 ·4H 2 O, 2 mM MgSO 4 ·7H 2 O, 5 mM HEPES and 12 mM N -acetyl- L -cysteine. After recovery for at least 2 h, the slices were transferred to a recording chamber mounted on an upright microscope (BX51WI, Olympus) equipped with IR-DIC optics. Slices were perfused with a carbogenated recording ACSF (at ~32 °C) containing 119 mM NaCl, 2.5 mM KCl, 4.0 mM CaCl 2 , 4.0 mM MgSO 4 , 1.0 mM NaH 2 PO 4 , 26.2 mM NaHCO 3 , 11 mM glucose, 5 mM HEPES and 0.1 mM picrotoxin. When measuring short-term facilitation of excitatory synapses onto OLM neurons, afferents in the SO were activated by a patch pipette that had a broken tip and was filled with recording ACSF, and EPSCs were recorded from OLM cells using a Multiclamp 700A (Molecular Devices). Recording patch electrodes were filled with an internal solution containing 135 mM caesium methanesulfonate, 10 mM HEPES, 0.2 mM EGTA, 8 mM NaCl, 4 mM Mg-ATP, 0.3 mM Na 3 GTP and 0.4% biocytin (pH 7.2 with CsOH, osmolarity adjusted to 285 mOsm). Data acquisition and analysis were performed using custom Igor Pro (WaveMetrics) software routines. When analysing short-term facilitation in CA1 pyramidal neurons, another stimulating glass electrode was also placed in the stratum radiatum (two-pathway experiments). Perforated patch recordings were performed to study LTP of EPSPs in OLM neurons [28] . A stock of gramicidin (150 mg ml −1 ) in DMSO was prepared freshly every 2 h and diluted to 1:1,000 in a K + -based internal solution composed of the following: 135 mM K gluconate, 10 mM HEPES, 0.2 mM EGTA, 10 mM KCl, 4 mM Mg-ATP, 0.3 mM Na 3 GTP, 0.4% biocytin and 5 mM QX-314 Cl (pH 7.2 with KOH, osmolarity adjusted to 270 mOsm). The tip of a recording electrode was filled with a gramicidin-free internal solution and backfilled with a gramicidin-containing solution. Afferents to the OLM cell were activated every 20 s by a stimulating electrode placed in the SO, and baseline EPSPs were recorded in current-clamp mode for at least 10 min. To induce LTP, the amplifier was switched to voltage-clamp mode, neurons were held at −70 mV, and TBS(four bursts of five pulses at 100 Hz with an interval of 250 ms) was applied 10 times every 20 s [28] . After LTP was induced with TBS, the amplifier was returned to current-clamp mode, and EPSP recordings were continued. When the perforated patch recordings were finished, the membrane was ruptured by negative pressure or current injection and whole-cell mode was maintained for about 10 min to allow the OLM cells to be fully loaded with biocytin. For post hoc identification of the recorded cells, slices were fixed overnight at 4 °C in a solution containing 4% PFA in phosphate buffer. The slices were then blocked with 2% normal donkey serum, 0.1% Triton X-100 in PBS for 1 h at room temperature, reacted with an anti-somatostatin antibody overnight, washed with PBS five times for 1 h each and reacted with an Alexa488-conjugated donkey anti-goat IgG antibody (Molecular Probes) and tetramethyl–rhodamine-conjugated streptavidin (Molecular Probes). Serial scans along the optical ( z ) axis were obtained for image analysis. Handling-induced seizure susceptibility Four to five mice were housed per cage and left undisturbed for 2 weeks before testing their susceptibility to seizures. On the day of testing, immediately after the cage was removed from the rack, each mouse was picked up by its tail and placed in a clean cage. The occurrence of seizure was determined by behavioural signs such as tonic–clonic convulsions, Straub tail, excessive salivation and loss of posture during the 2-min observation period. Drug-induced seizure susceptibility PTZ (Sigma) was dissolved in physiologic saline and administered intraperitoneally at a dose of 50 mg kg −1 to 6-month-old WT and KO mice. After the injection, each mouse was placed in a clear container and closely monitored for 10 min. An observer who was blind to the genotypes measured the latency to the first generalized seizure. EEG recording EEG recordings were performed with 7- to 8-month-old WT and KO mice as described previously [58] . Stainless steel screws (1.1 mm in diameter) that served as EEG electrodes were implanted over the somatosensory cortex (1.5 mm lateral to midline, 1.0 mm posterior to bregma) under 1.5% halothane anaesthesia with N 2 O:O 2 (3:2) ventilation 1 week before recording. A reference electrode was implanted on the cerebellum (at the midline, 2.0 mm posterior to lambda). Electromyography electrodes were placed 2–3 mm apart from the cervical region of the trapezius muscle. EEG and electromyography data were collected for 5 days. Behavioural analysis Behavioural analysis of adult WT and KO mice (4- to 5-month-old littermates) was performed as previously described [59] . Mice were single-housed 1 week before the start and during the behavioural analysis. The behavioural experiments were conducted during the light phase (10:00 hours to 19:00 hours). Experimenters were blind to genotype. Behavioural testing was performed in the following order: homecage activity test, open field test, light–dark box test, elevated plus maze test, startle response and prepulse inhibition test, hole board test, hot plate test, tail flick test. Human subjects and mutation analysis of ELFN1 Each participating patient or the parent signed an informed consent form as approved by the Ethics Committees of RIKEN Institute and participating institutions. All of the patients and control individuals examined in this study are Japanese, a population that has been reported to have little or negligible stratification [30] , [60] , [61] . We first carried out a resequencing analysis of exons and their flanking intronic regions, using 184 patients with epilepsy (male, 99; female, 85; mean onset age 9.9 years; range, 2–21 years), 316 with autism (male, 262; female, 53; mean age 12.7 years; range, 3–32 years) and 311 control subjects (more than 20 years old). Genomic DNA from the peripheral venous blood of affected and unaffected individuals was extracted with a QIAamp DNA Blood Midi Kit (Qiagen, Hilden, Germany). DNA for mutation screening was amplified with an illustra GenomiPhi V2 DNA Amplification Kit (GE Healthcare). We designed PCR primers to amplify all coding regions of ELFN1 (GenBank accession number, NM_001128636.2), and amplified genomic DNA by PCR with KOD-Plus (Toyobo). The PCR products were analysed by direct sequencing, using the ABI PRISM 3730xl Genetic Analyzer (Applied Biosystems). All novel mutations identified in amplified DNA by GenomiPhi were verified by sequencing of PCR products, using genomic DNA as a template. Primer sequences and PCR conditions are available on request. Missense mutations were found both in the patient group (9 single-nucleotide polymorphisms (SNPs)) and in controls (4 SNPs). Therefore, in a second step, we focused on 7 SNPs that were found only in the patient group ( Supplementary Table 2 ). These missense mutations were further SNP-typed for 2170 control subjects (male, 889; female 1281; mean age 42.4 years; range, 14–86 years), and 4 (A481V, R650C, D678N, R691W) were finally identified as SNPs present only in patients in this study. Statistics No statistical methods were used to predetermine sample sizes. However, our sample sizes are similar to those reported in previous reports. Data distribution was assumed to be normal, although this was not formally tested. Statistical analyses were conducted by using the SPSS statistical package (ver. 16.0, SPSS Japan, Tokyo, Japan) or Statcel3 software (OMS, Saitama, Japan). Parametric data were analysed by using the two-tailed unpaired Student’s t -test or Welch’s t -test after testing for equality of variance by the F -test. Non-parametric data were analysed using Mann–Whitney’s U -test. Differences were defined as statistically significant when P <0.05. How to cite this article : Tomioka, N. H. et al . Elfn1 recruits presynaptic mGluR7 in trans and its loss results in seizures. Nat. Commun. 5:4501 doi: 10.1038/ncomms5501 (2014).